Diacylglycerol mediates regulation of TASK potassium channels by Gq-coupled receptors The two-pore domain potassium (K2P) channels TASK-1 ( KCNK3 ) and TASK-3 ( KCNK9 ) are important determinants of background K + conductance and membrane potential. TASK-1/3 activity is regulated by hormones and transmitters that act through G protein-coupled receptors (GPCR) signalling via G proteins of the Gα q/11 subclass. How the receptors inhibit channel activity has remained unclear. Here, we show that TASK-1 and -3 channels are gated by diacylglycerol (DAG). Receptor-initiated inhibition of TASK required the activity of phospholipase C, but neither depletion of the PLC substrate PI(4,5)P 2 nor release of the downstream messengers IP 3 and Ca 2+ . Attenuation of cellular DAG transients by DAG kinase or lipase suppressed receptor-dependent inhibition, showing that the increase in cellular DAG—but not in downstream lipid metabolites—mediates channel inhibition. The findings identify DAG as the signal regulating TASK channels downstream of GPCRs and define a novel role for DAG that directly links cellular DAG dynamics to excitability. Diacylglycerol (DAG) is one of the best-studied second messengers of eukaryotic cells [1] . It is released by stimulus-induced activation of phospholipase C (PLC), which cleaves the minor plasma membrane phospholipid phosphatidylinositol-4,5-bisphosphate (PI(4,5)P 2 ) to produce DAG and inositol-1,4,5-trisphosphate (IP 3 ). The PLCβ isozymes are activated by G protein-coupled receptors that signal through the G q/11 subclass of Gα proteins (GqPCRs). PLCβ activation occurs by direct interaction with the Gα protein; β/γ subunits and increased intracellular Ca 2+ can also promote PLCβ activation [2] . As a membrane-resident messenger, DAG operates not only by binding to target proteins, but also by recruiting DAG-binding proteins to the membrane [1] , [3] . Besides the prototypical DAG effector, protein kinase C (PKC), there is a structural and functional diversity of high-affinity DAG effector proteins [1] , [4] . However, common to all of these effectors is that the DAG interaction is mediated by cysteine-rich C1 domains, which mediate recruitment to the plasma membrane or activate the protein [5] . Little is known about DAG effectors that do not use C1 domains. Some members of the canonical TRP cation channels (TRPC) can be activated by DAG. The binding site and the molecular mechanism of activation by DAG are unknown [6] . Beyond its function as a messenger in its own right, DAG is also a precursor in the stimulus-driven production of several signalling lipids, including phosphatidic acid (PA), the endocannabinoid 2-arachidonoylglycerol (2-AG), free arachidonic acid and their downstream metabolites [4] . The TWIK-related acid-sensitive K + channels, TASK-1 and TASK-3 (KCNK3 and KCNK9), constitute a subgroup of the two-pore domain (K2P) potassium channel family [7] . These channels function as background or ’leak’ channels that are open at resting potentials and thus provide a resting K + conductance that strongly contributes to setting the membrane potential. In excitable cells TASK channels control action potential threshold and spiking patterns [8] , [9] , [10] . TASK channels show a broad, yet selective expression pattern in many organs, including the central nervous system, peripheral chemoreceptors, vascular smooth muscle and cardiac muscle, and adrenal cortex [7] , consistent with the involvement in the regulation of a wide variety of physiological processes. TASK-1 and -3 channels are extensively modulated by physiological stimuli. A defining property of TASK channels is closure on extracellular acidification near physiological pH [11] . Moreover, they are inhibited by hormones and transmitters that signal through GqPCRs [12] , [13] , [14] , [15] . The resulting cellular depolarization is thought to regulate processes such as motor control [10] , [15] , [16] and aldosterone secretion [17] . The precise signal-transduction pathway downstream of GqPCRs that operates TASK inhibition has remained unresolved. Here we show that DAG is both sufficient for TASK channel inhibition and necessary for downregulation by GqPCRs. In contrast, downstream intermediates of DAG had no or only a minor impact on channel activity. The results uncover a new and possibly widespread signalling role for the prototypic lipid messenger DAG. As TASK channels lack the archetypical C1 DAG-binding domain thought to mediate most cellular effects of DAG [1] , [4] , these channels may provide a new paradigm for C1-independent DAG effector proteins. PLC is required for TASK channel inhibition Receptor-mediated inhibition of TASK has been proposed to result from either direct interaction with activated Gα q [18] or from the action of a messenger downstream of the activity of PLCβ [12] , [19] . To differentiate between both candidate pathways, we first addressed the requirement for PLCβ in GqPCR-dependent channel inhibition. We started by testing pharmacological inhibition of PLCβ by the widely used PLC inhibitor U73122 (ref. 20 ). Application of U73122 almost completely abrogated inhibition of TASK-3 channels in response to activation of the co-expressed Gq-coupled muscarinic M1 receptor (M1R) in Chinese hamster ovary (CHO) cells ( Fig. 1a–c ). The inactive analogue, U73343, had no effect on receptor-mediated channel inhibition. Because previously reported effects of U73122 on TASK regulation have been controversial [12] , [18] , [19] , [21] , [22] , we additionally controlled for the efficacy of U73122 under our experimental conditions. By using total internal reflection fluorescence microscopy (TIRF-M) measurements with the PI(4,5)P 2 -binding translocation sensor PLCδ1-PH-GFP as a readout for PLC activity [20] , [23] , [24] , we confirmed that PLCβ was essentially disabled by preapplication of U73122 ( Fig. 1d–f ). In this assay the TIRF signal amplitude directly reports the degree of sensor binding to the membrane, and thus the concentration of its ligand PI(4,5)P 2 . Therefore, fluorescence decrease indicates depletion of PI(4,5)P 2 and hence PLC activity. Pre-application of 5 μM U73122, but not U73343, prevented translocation of PLCδ1-PH-GFP from the membrane on activation of M1R. Equivalent results were obtained using a DAG sensor (PKCγ-C1-GFP [20] , [25] ) for detection of PLC activity (not shown). 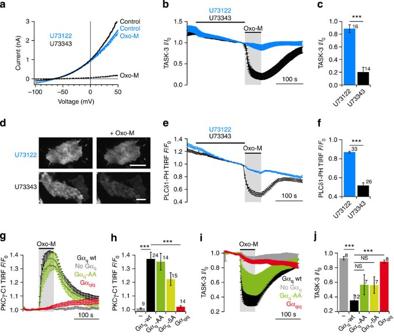Figure 1: Phospholipase C (PLC) is necessary for GqPCR-mediated TASK-3 inhibition. (a) PLC inhibitor U73122 disabled GqPCR-mediated inhibition of TASK-3. Representative K+currents from CHO cells co-transfected with hTASK-3 and M1R before (continuous) and after application of the muscarinic agonist, oxotremorine-M (Oxo-M, 10 μM for all experiments; dashed trace). Recordings were made following application of either 5 μM U73122 (blue) or the inactive analogue U73343 (black). (b) Average time course of TASK-3 currents at +50 mV from experiments as in (a). Currents were normalized to the amplitude immediately before application of Oxo-M. (c) Mean residual currents after application of Oxo-M. (d) Inhibition of PLCβ by U73122 was confirmed by the PI(4,5)P2sensor PLCδ1-PH-GFP. Representative TIRF images of CHO cells co-transfected with PLCδ1-PH-GFP and M1R before (left panels) and during application of 10 μM Oxo-M (right panels). Scale bar, 20 μm. (e) Mean time course of single-cell TIRF intensity normalized to fluorescence before application of Oxo-M. (f) Mean normalized TIRF intensity at the end of the Oxo-M application. (g) M1R-induced activity of PLC was measured in Gαq/11−/−fibroblasts co-transfected with DAG sensor PKCγ-C1-GFP, M1R, and either no Gαq, wild-type Gαq, mutant Gαq-AA or a Gαqiqchimera deficient in coupling to PLC. PLC activity was probed as the degree of membrane association of PKCγ-C1-GFP with TIRF microscopy. (h) Mean normalized increase in membrane association of PKCγ-C1-GFP at the end of the application of Oxo-M in the presence of Gαqor the mutant forms Gαq-AA, Gαq-5A or Gαqiq. (i,j) Differential inhibition of TASK-3 current by receptor activation in Gαq/11−/−fibroblasts when co-expressed with either wild type or mutant Gαq. Error bars indicate s.e.m. ***P<0.001; **P<0.01; *P<0.05. Numbers on bar graphs indicate the number of replicates (individual cells). Figure 1: Phospholipase C (PLC) is necessary for GqPCR-mediated TASK-3 inhibition. ( a ) PLC inhibitor U73122 disabled GqPCR-mediated inhibition of TASK-3. Representative K + currents from CHO cells co-transfected with hTASK-3 and M1R before (continuous) and after application of the muscarinic agonist, oxotremorine-M (Oxo-M, 10 μM for all experiments; dashed trace). Recordings were made following application of either 5 μM U73122 (blue) or the inactive analogue U73343 (black). ( b ) Average time course of TASK-3 currents at +50 mV from experiments as in ( a ). Currents were normalized to the amplitude immediately before application of Oxo-M. ( c ) Mean residual currents after application of Oxo-M. ( d ) Inhibition of PLCβ by U73122 was confirmed by the PI(4,5)P 2 sensor PLCδ1-PH-GFP. Representative TIRF images of CHO cells co-transfected with PLCδ1-PH-GFP and M1R before (left panels) and during application of 10 μM Oxo-M (right panels). Scale bar, 20 μm. ( e ) Mean time course of single-cell TIRF intensity normalized to fluorescence before application of Oxo-M. ( f ) Mean normalized TIRF intensity at the end of the Oxo-M application. ( g ) M1R-induced activity of PLC was measured in Gα q/11 −/− fibroblasts co-transfected with DAG sensor PKCγ-C1-GFP, M1R, and either no Gα q , wild-type Gα q , mutant Gα q -AA or a Gα qiq chimera deficient in coupling to PLC. PLC activity was probed as the degree of membrane association of PKCγ-C1-GFP with TIRF microscopy. ( h ) Mean normalized increase in membrane association of PKCγ-C1-GFP at the end of the application of Oxo-M in the presence of Gα q or the mutant forms Gα q -AA, Gα q -5A or Gα qiq . ( i , j ) Differential inhibition of TASK-3 current by receptor activation in Gα q/11 −/− fibroblasts when co-expressed with either wild type or mutant Gα q . Error bars indicate s.e.m. *** P <0.001; ** P <0.01; * P <0.05. Numbers on bar graphs indicate the number of replicates (individual cells). Full size image Previous work addressed the role of PLC by employing a double mutant of Gα q (Gα q -AA) thought to disable activation of PLC by active Gα q . When expressed in cells lacking both Gα q and Gα 11 (Gα q/11 −/− embryonic fibroblasts), Gα q -AA reconstituted TASK channel inhibition, thus questioning the role of PLC in TASK channel regulation [18] . However, by using PKCγ-C1-GFP as a sensor of PLC activity we found that when expressed in Gα q/11 −/− cells, Gα q -AA efficiently activated PLC on receptor stimulation with little difference to wild-type Gα q ( Fig. 1g,h ). Further introduction of additional three mutations reported to impair Gq/PLC-coupling (Gα q -5A) [26] only slightly affected PLC activation. Accordingly, both Gα q mutants restored receptor-mediated inhibition of TASK-3 in Gα q/11 −/− fibroblasts ( Fig. 1i,j ). Recently, Zhang et al. [27] developed a chimeric Gα q (Gα qiq ) in which the PLC interaction domain is replaced by the homologous region of Gα i . This construct can still be activated by GqPCRs, but coupling to PLC is abrogated. When Gα qiq was co-expressed with the M1R receptor and the PKCγ-C1 sensor domain in Gα q/11 -deficient cells, activation of PLC was lacking ( Fig. 1g,h ), confirming elimination of functional coupling to PLC. As shown in Fig. 1i,j , Gα qiq was unable to restore M1R-mediated inhibition of TASK-3 in Gα q/11 −/− fibroblasts. We therefore conclude that activation of PLC by Gα q is an indispensable step for the receptor-mediated inhibition of TASK channels. Intracellular Ca 2+ at or above the physiological resting concentrations is an established requirement for GqPCR-stimulated PLCβ activity [20] . We used this Ca 2+ dependence as an additional criterion for assessing the involvement of PLC. When intracellular Ca 2+ was clamped to values below physiological resting levels by inclusion of the Ca 2+ chelator BAPTA (20 mM) in the intracellular solution, PLC activity, as measured by translocation of the PKCγ-C1 sensor, was indeed abrogated. Receptor-mediated inhibition of TASK-3 channels measured simultaneously from the same cells was also entirely abolished ( Fig. 2a ). Similarly, 20 mM EGTA largely prevented inhibition of TASK, whereas 5 mM BAPTA only partially occluded channel inhibition ( Fig. 2b ), which is similar to previous findings showing that buffering with 5 mM BAPTA did not prevent TASK channel regulation [12] . As high buffer concentrations or extremely low intracellular Ca 2+ levels might also affect other cellular processes, we further tested for the effects of this condition on signalling upstream of PLC activity. To this end we used a FRET assay to monitor receptor-induced interaction between Gα q and PLCβ. As shown in Fig. 2c , the FRET signal between Gα q -CFP and YFP-PLCβ3 rapidly increased on activation of co-expressed M1R receptor, directly reporting the interaction. This increase in FRET was not disrupted by high intracellular BAPTA. Thus, upstream signalling including the function of Gα q remained functional, supporting the conclusion that the effect of BAPTA on TASK channel regulation resulted from inhibition of PLC. 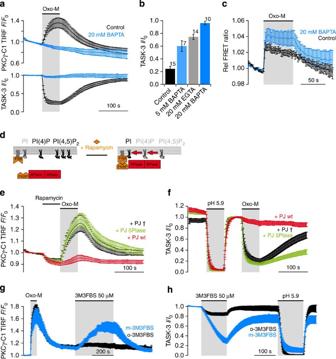Figure 2: Involvement of PLC in GqPCR-mediated TASK-3 inhibition. (a) Strong buffering of intracellular Ca2+suppressed TASK-3 inhibition by M1R. CHO cells co-expressing TASK-3, DAG sensor PKCγ-C1-GFP and M1R were whole-cell patch-clamped with intracellular solutions buffered to either 0.1 μM free Ca2+(control) or without Ca2+but 20 mM of the Ca2+chelator BAPTA. PKCγ-C1-GFP translocation was monitored simultaneously by TIRF microscopy. (b) Mean residual currents after application of 10 μM Oxo-M with either 0.1 μM intracellular Ca2+(control) or the Ca2+chelators indicated. (c) Dynamic FRET measurements between Gαq-CFP and YFP-PLCβ3 were done with whole-cell patch-clamped cells after 4 min of equilibration with solutions containing either 0.1 μM free Ca2+(control,n=9) or 20 mM BAPTA (n=9). Rapid increase in FRET following activation of co-expressed M1R indicates comparable association of Gαqand PLCβ3 in both conditions. (d) Principle of induced depletion of PLC substrate. Application of rapamycin triggers heterodimerization of FRB/FKBP, leading to irreversible recruitment of pseudojanin (PJ) to the plasma membrane. PJ comprises a 4-phosphatase and 5-phosphatase domain, degrading both PI(4,5)P2and PI(4)P. (e) PLC-mediated DAG production was blocked by recruitment of PJ (n=16), but not catalytically inactivated PJ (PJ†;n=24) or PJ with exclusive 5-phosphatase activity (PJ 5Ptase;n=36). Cells were co-transfected with PKCγ-C1-GFP, M1R, Lyn11-FRB and PJ variants fused to mcherry-FKBP. Cells were selected for membrane recruitment of mcherry. (f) Recruitment of PJ, (n=14), but not PJ-5Ptase (n=9) or catalytically inactive PJ† (n=12), suppressed current inhibition by M1R without affecting channel gating by extracellular acidification. Cells were co-transfected with TASK-3, M1R, Lyn11-FRB and PJ variants. Rapamycin (5 μM) was applied before the experiments shown. Cells were selected for membrane translocation of mcherry, or for PJ wt for translocation of co-expressed PLCδ1-PH-GFP, indicating depletion of PI(4,5)P2. (g) m-3M3FBS induced translocation of the DAG sensor PKCγ-C1-GFP, indicating reversible activation of PLC (n=20 cells from three experiments). The inactive analogue o-3M3FBS was largely ineffective (n=15 cells from three experiments). (h) Application of m-3M3FBS (n=9) but not o-3M3FBS (n=7) reversibly inhibited TASK-3 current. Error bars indicate s.e.m. Figure 2: Involvement of PLC in GqPCR-mediated TASK-3 inhibition. ( a ) Strong buffering of intracellular Ca 2+ suppressed TASK-3 inhibition by M1R. CHO cells co-expressing TASK-3, DAG sensor PKCγ-C1-GFP and M1R were whole-cell patch-clamped with intracellular solutions buffered to either 0.1 μM free Ca 2+ (control) or without Ca 2+ but 20 mM of the Ca 2+ chelator BAPTA. PKCγ-C1-GFP translocation was monitored simultaneously by TIRF microscopy. ( b ) Mean residual currents after application of 10 μM Oxo-M with either 0.1 μM intracellular Ca 2+ (control) or the Ca 2+ chelators indicated. ( c ) Dynamic FRET measurements between Gα q -CFP and YFP-PLCβ3 were done with whole-cell patch-clamped cells after 4 min of equilibration with solutions containing either 0.1 μM free Ca 2+ (control, n =9) or 20 mM BAPTA ( n =9). Rapid increase in FRET following activation of co-expressed M1R indicates comparable association of Gα q and PLCβ3 in both conditions. ( d ) Principle of induced depletion of PLC substrate. Application of rapamycin triggers heterodimerization of FRB/FKBP, leading to irreversible recruitment of pseudojanin (PJ) to the plasma membrane. PJ comprises a 4-phosphatase and 5-phosphatase domain, degrading both PI(4,5)P 2 and PI(4)P. ( e ) PLC-mediated DAG production was blocked by recruitment of PJ ( n =16), but not catalytically inactivated PJ (PJ†; n =24) or PJ with exclusive 5-phosphatase activity (PJ 5Ptase; n =36). Cells were co-transfected with PKCγ-C1-GFP, M1R, Lyn11-FRB and PJ variants fused to mcherry-FKBP. Cells were selected for membrane recruitment of mcherry. ( f ) Recruitment of PJ, ( n =14), but not PJ-5Ptase ( n =9) or catalytically inactive PJ† ( n =12), suppressed current inhibition by M1R without affecting channel gating by extracellular acidification. Cells were co-transfected with TASK-3, M1R, Lyn11-FRB and PJ variants. Rapamycin (5 μM) was applied before the experiments shown. Cells were selected for membrane translocation of mcherry, or for PJ wt for translocation of co-expressed PLCδ1-PH-GFP, indicating depletion of PI(4,5)P 2 . ( g ) m-3M3FBS induced translocation of the DAG sensor PKCγ-C1-GFP, indicating reversible activation of PLC ( n =20 cells from three experiments). The inactive analogue o-3M3FBS was largely ineffective ( n =15 cells from three experiments). ( h ) Application of m-3M3FBS ( n =9) but not o-3M3FBS ( n =7) reversibly inhibited TASK-3 current. Error bars indicate s.e.m. Full size image Although it had been suggested that depletion of the PLC substrate, PI(4,5)P 2 , may be the signal triggering channel deactivation [12] , [28] , we recently showed that depletion of PI(4,5)P 2 does not alter channel activity of TASK-1 and TASK-3 (ref. 29 ). Yet, the requirement for PLC implies an indirect role of its substrate PI(4,5)P 2 , as a sufficient concentration of substrate must be present to allow for the production of any downstream signalling intermediate. We therefore probed the regulation of TASK channels during forced depletion of PI(4,5)P 2 and its precursor PI(4)P by pseudojanin, an engineered chimeric phosphoinositide phosphatase that degrades PI(4,5)P 2 and PI(4)P [29] , [30] . Pseudojanin was acutely activated by recruitment to the membrane via rapamycin-dependent heterodimerization ( Fig. 2d ) [29] , [31] . Pseudojanin-mediated depletion of PI(4,5)P 2 and PI(4)P precluded PLC activity on subsequent activation of M1R as indicated by lack of DAG production ( Fig. 2e ) and abolished channel inhibition ( Fig. 2f ). As it was previously shown that transcriptional induction of a PI(4,5)P 2 5-phosphatase did not affect regulation of TASK currents by G q -coupled receptors [18] , we also tested for an effect of selective depletion of PI(4,5)P 2 . To this end we used a pseudojanin construct in which the PI(4)P 4-phosphatase SAC1 was inactivated by mutation (PJ-5Ptase). As shown in Fig. 2f , recruitment of PJ-5Ptase did not affect TASK regulation. However, monitoring the production of DAG under this condition revealed that the receptor-induced DAG transient was also unchanged ( Fig. 2e ). Thus, despite depletion of PI(4,5)P 2 , PLC activity is not reduced to a measurable degree. Selective activation of a 5-phosphatase may not be sufficient to lower PI(4,5)P 2 concentration enough to eliminate PI(4,5)P 2 turnover by PLC, perhaps because some PI(4,5)P 2 is continuously resynthesized from the augmented PI(4)P pool. Alternatively, PI(4)P may itself also be a relevant substrate of PLCβ [20] . In conclusion, the requirement of PI(4,5)P 2 and PI(4)P for TASK channel regulation by GqPCRs but not for basal channel activity corroborates the role of PLC activity in TASK regulation. We next asked whether PLC activity is also sufficient for inhibiting TASK channels. To this end, we used the benzenesulfonamide m-3M3FBS that activates PLC independent of GqPCRs [20] , [32] . According to plasma membrane translocation of the DAG sensor PKCγ-C1 m-3M3FBS, but not its inactive analogue o-3M3FBS, activated PLC when applied to CHO cells ( Fig. 2g ). The kinetics and amplitude of sensor translocation indicated that activation of PLC by m-3M3FBS occurred more slowly and was somewhat weaker compared with PLC activity triggered by M1R. As shown in Fig. 2h , application of m-3M3FBS robustly inhibited TASK-3 currents, whereas the inactive analogue had little effect. Current inhibition developed slowly, was slowly reversible and was less complete compared with receptor activation, mirroring the characteristics of PLC activation as monitored with the fluorescent sensor of PLC activity. Taken together, these data demonstrate that activation of PLCβ is an essential requirement for inhibition of TASK-3 channels by a G q -coupled receptor and that activation of PLC is sufficient to induce channel inhibition. Hence, the signal that mediates channel closure must be downstream of PLCβ. Diacylglycerol inhibits TASK channels To identify the relevant biochemical signal, we next directly applied candidate downstream messengers to TASK channels. Application of the membrane permeable short-chain DAG analogue 1,2-Dioctanoyl- sn -glycerol (DiC8) [25] to CHO cells expressing TASK-3 or TASK-1 resulted in dose-dependent and reversible current inhibition ( Fig. 3a,b ). At the same concentration range, DiC8 induced robust but sub-maximal translocation of the DAG sensor domain PKCγ-C1-GFP to the plasma membrane ( Fig. 3c ), suggesting that the concentrations reached by exogenous application may be comparable to cellular concentrations of endogenous DAG produced on stimulation of GqPCRs. 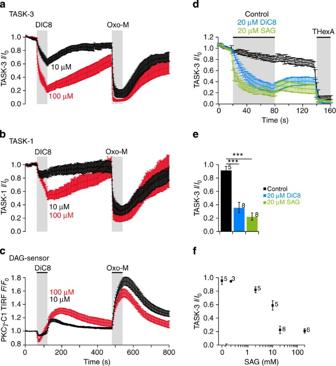Figure 3: DAG directly inhibits TASK-1 and -3 channels. (a) Application of short-chain DAG analogue (1,2-dioctanoyl-sn-glycerol; DiC8) onto CHO cells reversibly inhibited TASK-3;n=7 both for application of 10 μM (black) and 100 μM DiC8 (red). (b) Application of 10 μM (n=8) or 100 μM (n=6) DiC8 to CHO cells expressing TASK-1. (c) Membrane association of DAG sensor PKCγ-C1-GFP induced by application of DiC8 to CHO cells (10 or 100 μM;n≥29 cells from ≥6 experiments, each). Activation of the co-expressed M1R by 10 μM Oxo-M served as a control for strong DAG production. (d) Application of DiC8 and 1-Stearyl-2-arachidonoyl-sn-glycerol (SAG) inhibited TASK-3 channels when applied to the intracellular face of giant inside-out patches excised fromXenopusoocytes. Tetrahexylammonium (THexA; 10 μM) completely blocking the channel was applied to gauge overall TASK-3 currents. Shown are mean currents measured at +50 mV at the end of each repetitive voltage ramp, normalized to current size before application (t=30 s). (e) Residual TASK-3 currents at the end of the DAG application from experiments in (d). *** indicatesP<0.001. (f) Dose-dependent inhibition of TASK-3 currents by SAG, measured in giant patches as in (d,e). Data are presented as mean±s.e.m. Figure 3: DAG directly inhibits TASK-1 and -3 channels. ( a ) Application of short-chain DAG analogue (1,2-dioctanoyl- sn -glycerol; DiC8) onto CHO cells reversibly inhibited TASK-3; n =7 both for application of 10 μM (black) and 100 μM DiC8 (red). ( b ) Application of 10 μM ( n =8) or 100 μM ( n =6) DiC8 to CHO cells expressing TASK-1. ( c ) Membrane association of DAG sensor PKCγ-C1-GFP induced by application of DiC8 to CHO cells (10 or 100 μM; n ≥29 cells from ≥6 experiments, each). Activation of the co-expressed M1R by 10 μM Oxo-M served as a control for strong DAG production. ( d ) Application of DiC8 and 1-Stearyl-2-arachidonoyl- sn -glycerol (SAG) inhibited TASK-3 channels when applied to the intracellular face of giant inside-out patches excised from Xenopus oocytes. Tetrahexylammonium (THexA; 10 μM) completely blocking the channel was applied to gauge overall TASK-3 currents. Shown are mean currents measured at +50 mV at the end of each repetitive voltage ramp, normalized to current size before application ( t =30 s). ( e ) Residual TASK-3 currents at the end of the DAG application from experiments in ( d ). *** indicates P <0.001. ( f ) Dose-dependent inhibition of TASK-3 currents by SAG, measured in giant patches as in ( d , e ). Data are presented as mean±s.e.m. Full size image As shown in Fig. 3d,e , application of DiC8 to the cytoplasmic face of giant patches excised from Xenopus oocytes similarly inhibited TASK-3 activity. The effectiveness in this cell-free condition points to a direct action of DAG on the channel and argues against an involvement of DAG-dependent protein kinase (PKC) or of DAG metabolites. The inside-out configuration of the giant patch also allowed for the direct delivery of ‘native’ long-chain DAG to the inner leaflet of the membrane ( Fig. 3d-f ). Endogenous DAG produced by PLCβ is predominantly 1-stearoyl-2-arachidonoylglycerol (SAG) [33] . Application of SAG (20 μM) to giant patches produced a potent inhibition of TASK-3, with an efficacy slightly greater than the short-chain analogue DiC8 at the same concentration ( Fig. 3d,e ). Channel inhibition was dose-dependent with a half-inhibiting concentration of about 10 μM ( Fig. 3f ). Inhibition was poorly reversible, presumably because partitioning of SAG into the plasma membrane is not readily reversible. We further tested the lipid metabolites 2-arachidonoyl-glycerol (2-AG) derived from DAG by diacylglycerol lipases (DGLs), and phosphatidic acid (PA) generated by phosphorylation of DAG through diacylglycerol kinases (DGKs) [4] . Consistent with a previous report [34] , the endocannabinoid 2-AG also inhibited TASK-3, albeit with a lower efficacy compared with SAG ( Fig. 4a,b ). PA or arachidonic acid (AA), which can be released from 2-AG, had little effect on channel activity. 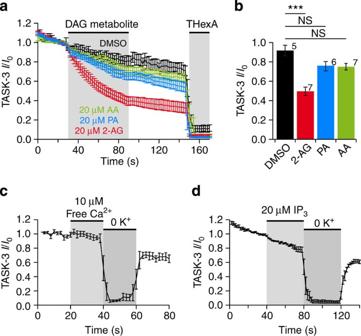Figure 4: DAG metabolites, IP3and intracellular Ca2+have little effect on TASK-3 channel activity. (a) Effects of DAG metabolites on TASK-3 currents in giant inside-out patches fromXenopusoocytes. Control data with application of vehicle (DMSO) is replotted fromFig. 3dfor comparison. (b) Mean residual TASK-3 currents measured at the end of the application of the various lipids from experiments in (a). (c) Application of 10 μM free Ca2+to the intracellular face of giant patches was without effect on TASK-3 currents (n=6). Currents measured as in (a). Subsequent removal of intracellular K+completely eliminated K+outward currents, verifying that currents were mediated by TASK-3. (d) Application of 20 μM IP3(n=7) to inside-out patches did not inhibit TASK-3 currents. Giants patch recordings were done as in (a) and (c). Data are presented as mean±s.e.m. Figure 4: DAG metabolites, IP 3 and intracellular Ca 2+ have little effect on TASK-3 channel activity. ( a ) Effects of DAG metabolites on TASK-3 currents in giant inside-out patches from Xenopus oocytes. Control data with application of vehicle (DMSO) is replotted from Fig. 3d for comparison. ( b ) Mean residual TASK-3 currents measured at the end of the application of the various lipids from experiments in ( a ). ( c ) Application of 10 μM free Ca 2+ to the intracellular face of giant patches was without effect on TASK-3 currents ( n =6). Currents measured as in ( a ). Subsequent removal of intracellular K + completely eliminated K + outward currents, verifying that currents were mediated by TASK-3. ( d ) Application of 20 μM IP 3 ( n =7) to inside-out patches did not inhibit TASK-3 currents. Giants patch recordings were done as in ( a ) and ( c ). Data are presented as mean±s.e.m. Full size image Application of either IP 3 or Ca 2+ to TASK-3 had no effect on channel activity ( Fig. 4c,d ), indicating that the IP 3 /Ca 2+ branch of the PLC-dependent signal-transduction cascade is not involved in TASK regulation by GqPCRs. DAG dynamics mediate receptor-induced TASK inhibition These results indicated DAG as a likely messenger mediating TASK channel modulation. We therefore asked whether DAG indeed mediates channel inhibition in response to GqPCR activity. We aimed at altering cellular DAG dynamics and reasoned that accelerating the turnover of DAG should reduce the DAG concentrations reached on receptor stimulation. Cellular DAG accumulating on activation of PLCβ is cleared by DGKs or by DGLs [4] . Among the 12 isoforms of DGK we found DGKβ to be constitutively localized at the plasma membrane when overexpressed in CHO cells ( Fig. 5a inset), suggesting that it may effectively turn over DAG after receptor activation. Indeed, expression of DGKβ strongly blunted the receptor-induced DAG transient in CHO cells ( Fig. 5a,c ). When co-expressed with TASK-3 channels, DGK similarly suppressed channel inhibition by activation of M1R ( Fig. 5d,f ). Overexpression of DAG lipase alpha (DGLα [35] ) also strongly attenuated the receptor-induced accumulation of DAG ( Fig. 5b,c ). As shown in Fig. 5e,f , DGLα also suppressed receptor-mediated channel inhibition and accelerated current recovery when co-expressed with TASK-3 channels. 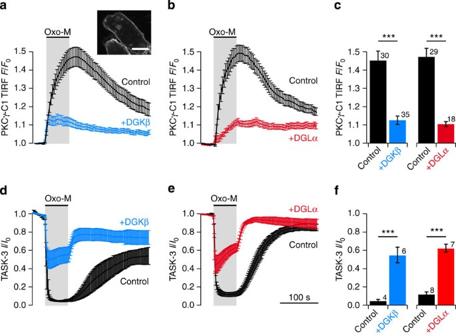Figure 5: Suppression of cellular DAG-transients attenuates receptor-mediated TASK-3 inhibition. (a) DAG concentration dynamics in CHO cells induced by M1R (10 μM Oxo-M) were measured by TIRF microscopy of PKCγ-C1-GFP either in the absence (control) or with co-expression of DAG-kinase β (DGKβ). Confocal image (inset) shows membrane localization of GFP-tagged DGKβ (Scale bar, 10 μm). (b) Receptor-induced DAG dynamics measured as in (a) either without (control) or with co-expression of DAG lipase α (DGLα). (c) Mean TIRF signal increase (± s.e.m.) at the end of 60 s Oxo-M application from experiments shown in (a) and (b). Numbers indicate individual recordings. (d) TASK-3 current inhibition by activation of M1R with or without co-expression of DGKβ. (e) TASK-3 current inhibition by activation of M1R with or without co-expression of DGLα. (f) Mean residual TASK-3 currents at the end of Oxo-M application from the experiments shown in (d,e). Current inhibition was strongly reduced by either DGKβ or DGLα, matching the suppressed DAG transients (a–c). Figure 5: Suppression of cellular DAG-transients attenuates receptor-mediated TASK-3 inhibition. ( a ) DAG concentration dynamics in CHO cells induced by M1R (10 μM Oxo-M) were measured by TIRF microscopy of PKCγ-C1-GFP either in the absence (control) or with co-expression of DAG-kinase β (DGKβ). Confocal image (inset) shows membrane localization of GFP-tagged DGKβ (Scale bar, 10 μm). ( b ) Receptor-induced DAG dynamics measured as in ( a ) either without (control) or with co-expression of DAG lipase α (DGLα). ( c ) Mean TIRF signal increase (± s.e.m.) at the end of 60 s Oxo-M application from experiments shown in ( a ) and ( b ). Numbers indicate individual recordings. ( d ) TASK-3 current inhibition by activation of M1R with or without co-expression of DGKβ. ( e ) TASK-3 current inhibition by activation of M1R with or without co-expression of DGLα. ( f ) Mean residual TASK-3 currents at the end of Oxo-M application from the experiments shown in ( d , e ). Current inhibition was strongly reduced by either DGKβ or DGLα, matching the suppressed DAG transients ( a – c ). Full size image These findings are consistent with DAG acting as the endogenous messenger that inhibits TASK channels. At the same time, the results rule out a major role of downstream lipid messengers in inhibiting TASK channels, including PA and 2-AG and its metabolites, as their concentrations should be increased rather than decreased by DGK and DGL, respectively. We note that the impairment of current inhibition by DGLα appears less pronounced than the decrease in the DAG transient reported by the PKCγ-C1-GFP sensor. However, the remaining channel inhibition may be readily explained by weak inhibition of TASK by the DGL product 2-AG, as observed in isolated patches ( Fig. 4a ). A proximal C-terminal motif essential for inhibition by DAG A six-amino-acid motif (VLRFLT) located at the proximal C terminus of TASK-3 channels is essential for the channels’ sensitivity to GqPCR modulation [14] . If DAG mediates the receptor’s effect, the same motif must also determine the sensitivity to exogenous DAG. We therefore next examined TASK channels with mutation or deletion of the short motif ( Fig. 6a ). 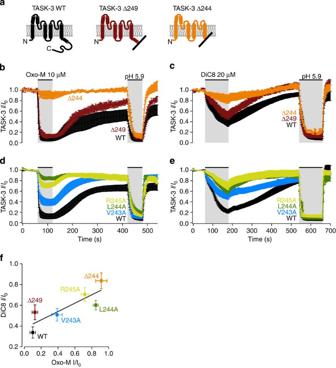Figure 6: The C-terminal VLRFLT motif is critical for DAG-mediated channel inhibition. (a) Schematic representation of C-terminal channel truncations: TASK-3 was truncated either after position 248, retaining the VLRFLT motif, (TASK-3 Δ249) or after position 243, removing the entire C terminus (TASK-3 Δ244). (b) Removal of the VLRFLT motif rendered TASK-3 currents insensitive to co-expressed Gq-coupled M1R, whereas truncation after this motif had no effect on channel regulation (n=6, 7 and 5 cells, for wt, Δ249, and Δ244 channels, respectively). Inhibition by extracellular acidification demonstrated that currents were carried by TASK-3 and confirmed functional integrity of truncated channels. (c) Whole-cell recordings of the effect of DiC8 on TASK-3 and truncated channels (n=9, 9 and 7 cells, for wt, Δ249 and Δ244 channels, respectively) expressed in CHO cells. (d) Point mutations in the VLRFLT motif reduced the channel sensitivity towards M1R-mediated inhibition (n=11, 10, 10, 11 cells for wt, V243A, L244A and R245A, respectively). (e) Channel mutants with attenuated receptor-induced inhibition also showed reduced sensitivity towards application of 20 μM DiC8 (n=5, 7, 7 and 5 cells for wt, V243A, L244A and R245A, respectively). (f) Correlation of channel inhibition by M1R receptor versus application of DiC8, derived from the experiments presented in (b–e). Shown are normalized current amplitudes at the end of the application of Oxo-M or DiC8 (mean±s.e.m.). Figure 6b shows that truncation of the C terminus of TASK-3 preserving the VLRFLT motif (Δ249) yielded functional channels still sensitive to regulation by GqPCRs, consistent with previous findings [14] . However, additional removal of the VLRFLT motif (Δ244) rendered the channel insensitive to activation of the co-expressed receptor. These channels were still gated by extracellular pH, indicating that the fundamental function of the truncated channels was not compromised. Strikingly, the sensitivity of these truncated channels to DAG mirrored their inhibition by the GqPCR. Thus, inhibition by DiC8 (20 μM) was unchanged in Δ249, but was abrogated by truncation of the VLRFLT motif ( Fig. 6c ). Figure 6: The C-terminal VLRFLT motif is critical for DAG-mediated channel inhibition. ( a ) Schematic representation of C-terminal channel truncations: TASK-3 was truncated either after position 248, retaining the VLRFLT motif, (TASK-3 Δ249) or after position 243, removing the entire C terminus (TASK-3 Δ244). ( b ) Removal of the VLRFLT motif rendered TASK-3 currents insensitive to co-expressed G q -coupled M1R, whereas truncation after this motif had no effect on channel regulation ( n =6, 7 and 5 cells, for wt, Δ249, and Δ244 channels, respectively). Inhibition by extracellular acidification demonstrated that currents were carried by TASK-3 and confirmed functional integrity of truncated channels. ( c ) Whole-cell recordings of the effect of DiC8 on TASK-3 and truncated channels ( n =9, 9 and 7 cells, for wt, Δ249 and Δ244 channels, respectively) expressed in CHO cells. ( d ) Point mutations in the VLRFLT motif reduced the channel sensitivity towards M1R-mediated inhibition ( n =11, 10, 10, 11 cells for wt, V243A, L244A and R245A, respectively). ( e ) Channel mutants with attenuated receptor-induced inhibition also showed reduced sensitivity towards application of 20 μM DiC8 ( n =5, 7, 7 and 5 cells for wt, V243A, L244A and R245A, respectively). ( f ) Correlation of channel inhibition by M1R receptor versus application of DiC8, derived from the experiments presented in ( b – e ). Shown are normalized current amplitudes at the end of the application of Oxo-M or DiC8 (mean±s.e.m.). Full size image We further analysed the relevance of this motif by replacing individual amino acids by alanine. As shown in Fig. 6d , these mutations impaired GqPCR-dependent regulation to different degrees, with the most pronounced effects observed in the L244A and R245A mutants. When challenged with DiC8, the resulting channel inhibition of L244A and R245A was also largely reduced ( Fig. 6e ). Overall, inhibition by DiC8 of the various mutant channels correlated well with their sensitivity to receptor activity ( Fig. 6f ). In conclusion, inhibition of TASK channels by DAG relies on the same molecular determinants that govern inhibition by Gq signalling, lending further support to the conclusion that receptor/Gq-induced TASK channel inhibition is mediated by increased DAG levels. DAG inhibits TASK currents in cerebellar granule neurons Regulation of TASK channels by Gq-coupled receptors strongly impacts on membrane potential and excitability in many cell types. In cerebellar granule neurons (CGNs), a large ‘standing outward’ current (IK SO ) dominated by TASK-1 and TASK-3 channels [36] , [37] , [38] controls resting potential and action potential firing [8] , [36] , [38] . Gq-coupled neurotransmitter receptors (including muscarinic acetylcholine receptors and metabotropic glutamate receptors) dynamically regulate CGN excitability by inhibition of TASK channels [12] , [39] . We examined the activity of short-chain DAG, DiC8, on IK SO in dissociated cultured CGNs. Application of DiC8 (100 μM) reduced the outward current by about 50%, similar to current suppression by extracellular acidification or activation of endogenous muscarinic acetylcholine receptors ( Fig. 7a,b ). As CGNs express other K2P channels in addition to TASK [40] , we combined extracellular acidification with application of DAG to test whether the DAG-sensitive currents correspond to neuronal TASK channels. As shown in Fig. 7c , only a minor fraction of residual IK SO remained sensitive to DAG when TASK currents were blocked by pH 5.9 and acid-sensitive TASK currents remained closed when switching back to pH 7.4 after exposure to DAG. These observations support the conclusion that most of the DAG-sensitive currents in CGNs was indeed mediated by TASK. Taken together, these findings suggest that the current component carried by TASK channels is sensitive to DAG, consistent with the idea that the inhibition of native TASK channels by neuronal GqPCRs is indeed mediated by DAG. 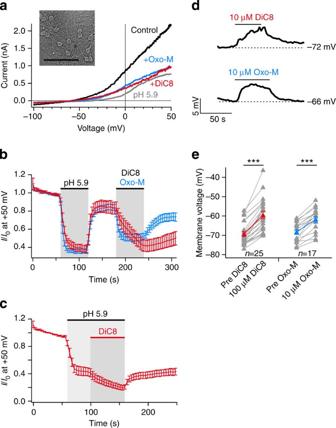Figure 7: Inhibition of native IKSOin cerebellar granule cells by DAG. (a) Representative whole-cell currents from a dissociated cerebellar granule cell (inset; scale bar, 50 μm). Currents were recorded in response to voltage ramps from a holding potential of +50 mV. Application of 10 μM Oxo-M to activate endogenous muscarinic receptors or 100 μM DiC8 inhibited outward potassium currents to a similar extent as extracellular acidification to pH 5.9. (b) Mean time course of standing outward currents during application of 10 μM Oxo-M (n=18) or 100 μM DiC8 (n=7), and extracellular acidification. Currents were measured at+50 mV and normalized to current amplitude before initial acidification. (Error bars indicate s.e.m.). (c) Mean time course of IKSOin response to combined application of low extracellular pH and DiC8 (100 μM). (d) Representative recordings of membrane potential during application of DiC8 (upper trace) or Oxo-M (lower trace). (e) Change of membrane potential induced by application of DiC8 (ΔVm=9.9±0.9 mV) or muscarinic receptor stimulation (ΔVm=6.5±0.8 mV) from experiments performed as in (d). *** indicatesP<0.001 tested with a paired Student’st-test. Figure 7: Inhibition of native IK SO in cerebellar granule cells by DAG. ( a ) Representative whole-cell currents from a dissociated cerebellar granule cell (inset; scale bar, 50 μm). Currents were recorded in response to voltage ramps from a holding potential of +50 mV. Application of 10 μM Oxo-M to activate endogenous muscarinic receptors or 100 μM DiC8 inhibited outward potassium currents to a similar extent as extracellular acidification to pH 5.9. ( b ) Mean time course of standing outward currents during application of 10 μM Oxo-M ( n =18) or 100 μM DiC8 ( n =7), and extracellular acidification. Currents were measured at+50 mV and normalized to current amplitude before initial acidification. (Error bars indicate s.e.m.). ( c ) Mean time course of IK SO in response to combined application of low extracellular pH and DiC8 (100 μM). ( d ) Representative recordings of membrane potential during application of DiC8 (upper trace) or Oxo-M (lower trace). ( e ) Change of membrane potential induced by application of DiC8 (Δ V m =9.9±0.9 mV) or muscarinic receptor stimulation (Δ V m =6.5±0.8 mV) from experiments performed as in ( d ). *** indicates P <0.001 tested with a paired Student’s t -test. Full size image Application of DAG also depolarized the membrane potential of CGNs by about 10 mV ( Fig. 7d,e ), similar to activation of endogenous ACh receptors, indicating that DAG-mediated regulation of TASK channels underlies modulation of neuronal electrical excitability. Here, we show that GqPCRs inhibit TASK channels through the production of DAG. Thus, several independent assays indicated that PLC activity is essential for channel inhibition. Among the downstream messengers of PLC, only DAG induced channel inhibition. Moreover, accelerating the turnover of DAG by overexpression of either DGK or DGL suppressed channel inhibition, demonstrating that liberation of DAG is indeed necessary for channel regulation. TASK channels are inhibited by DAG and not through messengers downstream of DAG, as DAG application rapidly inhibited channels in a cell-free system (excised patch), where recruitment of cytoplasmic DAG effectors, activation of kinase signalling, or conversion of DAG to downstream messengers is unlikely. In principle DAG could act on TASK channels via activation of protein kinase C (PKC), as pharmacological activation PKC can modulate TASK channels [41] . However, several careful studies consistently found that PKC does not mediate GqPCR-induced inhibition. Thus, neither removal of all potential PKC phosphorylation sites [14] , [41] nor pharmacological blockade of PKC [12] , [19] , [22] , [41] affected receptor-dependent channel regulation. This is in line with our current results showing that DAG is effective in isolated patches and inhibits truncated channels lacking potential PKC phosphorylation sites. The model that follows is direct binding of DAG to the channel. This could be binding of DAG directly either to the pore-forming α-subunits or to an accessory protein that is present in the plasma membrane and interacts with the α-subunit. We consider direct binding to the channel as the more simple and straightforward model, since (i) to our knowledge, appropriate interaction partners of TASK-1/3 are not known, (ii) the C-terminally truncated TASK channel should be deprived of much of its potential cytoplasmic protein–protein interaction interfaces and (iii) a relevant accessory protein would have to be ubiquitously and abundantly expressed in plasma membranes as DAG was effective in a wide variety of cells ranging from Xenopus oocytes to neurons; in fact, GPCR-mediated TASK channel inhibition is reported to work in essentially any cell type examined. As enzymatic conversion of DAG into PA or 2-AG reduced channel inhibition, these downstream intermediates cannot mediate channel inhibition. It is worth noting, however, that in the excised patch, 2-AG also inhibited TASK channels and that increased conversion of DAG to 2-AG did not fully block receptor-induced channel inhibition, although the DAG transient was strongly attenuated. Thus, production of 2-AG may also make a minor contribution to TASK channel regulation by GqPCRs. It was proposed previously that TASK inhibition is mediated by direct interaction with activated Gα q rather than by downstream signals [18] . In particular a direct biochemical interaction between Gα q and the TASK channel supports such a mechanism. However, as the various independent approaches blocking PLC function all abolished receptor-dependent inhibition it seems highly unlikely that Gα q alone could be sufficient to inhibit TASK channels. On the contrary, DAG by itself is sufficient to downregulate the channels. Yet it remains possible that Gα q could contribute to channel inhibition by increasing DAG affinity or efficacy through direct TASK-Gα q interaction, although such a model is speculative at present. Although the control of TASK-1/3 by DAG has not been recognized before, it is well established that other lipid compounds inhibit these channels. The endocannabinoid anandamide and its synthetic analogue methanandamide potently inhibit TASK channels by direct interaction with the channel [34] , [42] . Our current finding of partial inhibition by 2-AG suggests another endocannabinoid as a regulator of these background channels. Notably, all these compounds are chemically similar to DAG in consisting of arachidonic acid bound to a small moderately polar headgroup containing a hydroxyl group. It thus seems likely that all of these compounds share a common mechanism of TASK inhibition. It is further interesting to note that sanshool, the pungent compound of Szechuan pepper, acts by inhibiting TASK channels [43] . Sanshool is chemically similar to the aforementioned compounds in being an amide of a polyunsaturated fatty acid and a moderately polar alcohol. It is tempting to speculate that sanshool elicits sensory effects by hijacking a binding site at TASK channels built for regulation via endogenous lipid messengers. All well-characterized DAG effectors are earmarked by containing at least one prototypical C1 DAG-binding domain. Among the C1-containing proteins, the PKCs are often considered as the canonical and most important DAG effectors. Additional protein families containing C1 domains are the chimaerins, DGKs, protein kinase D and Munc13s [1] , [4] . In contrast, TASK channels do not contain a C1 domain. DAG also contributes to the activation of certain canonical TRP (TRPC) channels [6] , [44] , which also lack a C1 domain. To our knowledge, the binding site for DAG has not been identified. Our data show that a six-amino-acid motif (VLRFLT) at the most proximal intracellular C terminus of TASK-3 is crucial for DAG inhibition. Although its location close to the membrane’s inner leaflet may suggest a role in DAG binding, the membrane-proximal C terminus is implicated in gating of other K2P channels by a variety of stimuli. In TREK channels it mediates channel gating by phospholipids, membrane tension, intracellular pH and the antidepressant fluoxetine [45] , [46] , [47] . In TASK channels, the VLRFLT motif is also essential for channel activation by volatile anaesthetics [14] . Thus, it seems that the VLRFLT motif is most likely a gating element coupling DAG binding to channel closure; however, it is also possible that it contributes to binding of DAG. Yet, it remains to be shown if DAG indeed binds directly to the channel’s pore-forming subunit. If so, the fact that even the truncated minimalistic channel remains sensitive to DAG should facilitate identification of the DAG binding sites in TASK channels; the only intracellular structures to be considered as potential interaction sites of the headgroup of membrane-embedded DAG remaining in truncated TASK channel are the VLRFLT motif, a short N terminus of seven amino acids, and an intracellular loop of some 30 amino acids connecting M2 and M3. Thus, TASK channels may be amenable to the study of structural details of DAG binding and may serve as a novel paradigm for DAG effector molecules not operated via C1 domains. How might DAG alter gating to close the channels? Ashmole et al. [48] hypothesize that the underlying gating mechanism may be related to the gating by voltage, where depolarization increases open probability. Future single channel studies may provide more insights into the mechanistic details. Our results establish the control of K2P channels as a novel signalling role for DAG. Given the widespread expression of TASK channels and their established functions [7] , for example, in neurons [9] , [15] , [38] and adrenocortical cells [17] , this new signalling pathway is most likely important in many physiological processes. The tight regulation of plasma membrane DAG concentrations may be critical for maintaining appropriate TASK channel activity. Specifically, DAG concentration dynamics triggered by PLC activation depend on the rate of DAG clearance. Among the 10 mammalian DGK isoforms, several have been associated with the control and termination of PLC/DAG signalling in the plasma membrane [4] , [49] . Interestingly, mutation of DGKδ, one of DGK isoforms prominently expressed in the brain, is associated with epilepsy in humans and mice [50] . In principle, such a phenotype might result from excessive suppression of a potassium conductance by increased DAG levels. Knock-out of other neuronal DGKs also leads to neuronal and behavioural alterations that are linked to changed DAG signalling [51] , [52] . It should be interesting to examine whether dysregulation of TASK channel activity plays a role in these pathologies. DAG is also turned over by DGLs to generate the endocannabinoid 2-AG. Although their signalling function has been considered mostly in terms of production of the signalling lipids 2-AG and AA [35] , a role in regulating TASK channels by curtailing DAG signals should be considered, given that experimental overexpression of DGLα strongly affected DAG transients ( Fig. 5 ). In summary, our findings indicate that DAG dynamics and homeostasis directly control a multitude of cellular processes dependent on membrane potential, such as neuronal excitability, muscle contraction and hormone secretion through the inhibition of TASK-1 and -3 channels. Cell culture CHO dhFr − cells were grown at 37 °C with 5% CO 2 in minimum essential medium (MEM)-α with nucleosides supplemented with 10% fetal calf serum (Biochrom AG, Berlin, Germany), 100 U ml −1 penicillin and 100 μg ml −1 streptomycin. Gα q/11 −/− fibroblasts (kindly provided by Douglas A. Bayliss) were cultured at 37 °C with 5% CO 2 in Dulbecco’s modified eagle medium (DMEM) with high glucose and GlutaMax supplemented with 10% fetal calf serum (Biochrom AG), 100 U ml −1 penicillin and 100 μg ml −1 streptomycin. Both cell lines were seeded onto glass coverslips or glass-bottom dishes (WillCo Wells B.V., Amsterdam, The Netherlands) for electrophysiology and imaging experiments, respectively. One to two days after seeding cells were transfected using JetPEI (Polyplus Transfection, Illkirch, France) according to the manufacturer’s protocol. Experiments were performed 24–72 h post transfection. CGNs were prepared from P6-P9 Wistar rats. Animals were anaesthetized and decapitated to obtain cerebella, which were washed in ice-cold PBS, cut in 3–4 pieces and incubated at 37 °C for 15 min in 0.05% trypsin-EDTA/HBSS. After washing with DMEM, cerebelli were incubated with 10% DNase I (Sigma-Aldrich, Taufkirchen, Germany)/DMEM at 37 °C for 4 min. Cells were then triturated using fire-polished glass Pasteur pipettes with decreasing openings, passed through a 70-μm cell strainer and washed in a centrifugation step of 10 min at 210 g at 4 °C. CGNs were resuspended in DMEM with high glucose and GlutaMax supplemented with 10% horse serum (Biochrom AG), 100 U ml −1 penicillin and 100 μg ml −1 streptomycin and 25 mM KCl and plated on poly- D -lysine coated (MW 70,000-150,000; Sigma-Aldrich) glass coverslips with a density of 400,000 cells per cm 2 . After 1 h of cell sedimentation, 1 μM cytosine β- D -arabinofuranoside (Sigma-Aldrich) was added to the medium to prevent glial growth. Neurons were used for whole-cell recordings after 7–12 days in culture. Media and buffers used for cell culture were obtained from Gibco (Life Technologies, Carlsbad, CA, USA) unless noted otherwise. Molecular biology The following expression plasmids were used for transient transfection of CHO cells or Gα q/11 −/− fibroblasts: rat PKCγ-C1 (AA 26-89 in pEGFP-N1 NM_012628.1; obtained from Tobias Meyer); human PLCδ1-PH (AA 1-170 in pEGFP-N1; NM_006225.3, obtained from Tamas Balla); mouse Gα q (in pcDNA3, CFP inserted between AA 124/125 (ref. 53 ); NM_008139.5); mutant Gα q constructs Gα q -AA and Gα q -5A contain the point mutations R256A/T257A or DNE243-245AAA/R256A/T257A, respectively; human Gα qiq (chimera of Gαq AA 1-245+AA 333-359; NM_002072.4 and Gαi AA 242-328; NM_002070.3 in pcDNA3.1; kind gift from Xuming Zhang); human TASK-1 (in pcDNA3.1; NM_002246.2), human TASK-3 (in pcDNA3.1; NM_001282534.1; obtained from Jürgen Daut); human M1 receptor (in pSGHV0; NM_000738.2), rat DGKβ (in pEGFP-C3, GFP was removed for TIRF experiments; NM_019304.1, kindly provided by Fumio Sakane); human DGLα-GFP (in pcDNA3.1/V5-His TOPO; NM_006133.2, gift from Patrick Doherty); mcherry-FKBP-Pseudojanin (in pEGFP-C1; AA 30-108 of FKBP NM_054014.3, AA 2-517 of SAC1 NM_001179777.1, AA 214-644 of InPP5E NM_019892.4) [29] , [30] ; and Lyn11-FRB (in pC4RHE, AA 1-11 of Lyn11 (GCIKSKGKDSAGA), AA 2026-2121 of FRB NM_004958.3). Mutations of Gα q , hTASK-3, Pseudojanin (C392S of original SAC1) and C-terminal truncations of hTASK-3 were generated using the QuikChange II XL Site-Directed mutagenesis kit (Stratagene, Agilent Technologies, Waldbronn, Germany). For expression in oocytes, human TASK-3 in pSGEM was used. YFP was fused to the N terminus of human PLCβ3 via a 10 AS flexible linker by means of gateway cloning, and the resulting cDNA was cloned into pcDNA3. All constructs were verified by sequencing. Chemicals DAG analogues and metabolites (Avanti Polar Lipids, Alabaster, AL, USA) were prepared as 20 mM stock in DMSO. PLC inhibitor U73122 and the inactive analogue U73343 (Sigma-Aldrich) were prepared as 5 mM stock solution in DMSO, kept at −20 °C and diluted into physiological solutions <1 h before experiments. The PLC activator m-3M3FBS and its inactive analogue o-3M3FBS (Tocris Bioscience, Bristol, United Kingdom) were prepared as 50 mM stocks in DMSO. Muscarinic agonist Oxotremorine M (Oxo-M; Tocris Bioscience) was dissolved as 10 mM stock in water. Rapamycin was purchased as 5 mM solution in DMSO (Calbiochem, Merck Chemicals GmbH, Schwalbach, Germany). All drugs were stored at −20 °C and diluted in extracellular solution directly before usage. Inositol-1,4,5-trisphosphate (IP 3 ; Sigma-Aldrich) was prepared as 5 mM in water and diluted in intracellular solution for excised patch measurements. Patch-clamp Whole-cell voltage clamp experiments on CHO dhFr − , Gα q/11 −/− fibroblasts or primary CGNs were performed with an Axopatch 200B amplifier (Molecular Devices, Sunnyvale, CA, USA) controlled by PatchMaster v2x41 software (HEKA, Lambrecht/Pfalz, Germany) via an ITC-16 interface (InstruTECH, HEKA). Currents were low-pass filtered at 2 kHz and sampled at 5 kHz. Patch pipettes were pulled with a Sutter P-2000 (Sutter Instruments, Novato, CA, USA) from borosilicate glass (Science Products, Hofheim, Germany) to an open pipette resistance of 1.5 to 3 MΩ when filled with pipette solution containing (mM) 135 KCl, 5 Hepes, 5 EGTA, 3.5 MgCl 2 , 2.5 Na 2 ATP, 2.41 CaCl 2 and 0.1 Na 2 GTP, adjusted to pH 7.3 with KOH. To buffer intracellular Ca 2+ to effectively zero, the solutions contained (in mM) 85 KCl, 5 Hepes, 20 K 4 EGTA or K 4 BAPTA, 1 MgCl 2 , 2.5 Na 2 ATP and 0.1 Na 2 GTP. Alternatively, intracellular solution contained 5 mM K 4 BAPTA with KCl changed to 130 mM. Whole-cell serial resistance was <8 MΩ, which was compensated by 60%. Extracellular solution was composed of (mM) 144 NaCl, 10 HEPES, 5.8 KCl, 5.6 glucose, 1.3 CaCl 2 , 0.9 MgCl 2 , 0.7 NaH 2 PO 4 and set to pH 7.4 or pH 8.4 (for TASK-1) or pH 5.9 (to block TASK currents) with NaOH. Owing to the development of a cationic current during application of U73122, the extracellular Na + was substituted with NMDG + in the respective recordings. Giant patch recordings from Xenopus laevis oocytes were performed as described previously [54] . In brief, cRNA was synthesized using the mMESSAGE mMACHINE Kit (Ambion, Life Technologies). Xenopus laevis oocytes were obtained from EcoCyte Bioscience (Castrop-Rauxel, Germany). Following injection of cRNA, oocytes were incubated at 18 °C for 1–3 days before performing giant patch recordings. Currents were recorded using an EPC10 amplifier (HEKA) controlled by PatchMaster (HEKA), low-pass filtered at 2.9 kHz and sampled at 5 kHz. Giant patch pipettes were fire-polished to obtain open pipette resistances of 0.2–0.5 MΩ when filled with extracellular solution containing (mM) 115 NaCl, 10 HEPES, 5 KCl, 1.5 CaCl 2 , 1 MgCl 2 , adjusted to pH 7.4 with NaOH. Patches were excised into intracellular bath solution containing (in mM) 120 KCl, 5 HEPES, 3.5 MgCl 2 , 1 K 2 EGTA and was set to pH 7.2 with KOH. Intracellular solutions were applied to the cytoplasmic face of the patch with a multi-barrel gravity-driven application system. For K + -free intracellular solution 120 mM NaCl was substituted for KCl. For application of intracellular Ca 2+ , the K 2 EGTA concentration was reduced to 2 mM and 1.98 mM Ca 2+ was added, yielding 10 μM free Ca 2+ . In these experiments chloride was substituted by methanesulfonate to minimize currents through Ca 2+ -activated chloride channels. All recordings were performed at room temperature (~21 °C). TASK currents were recorded in response to voltage ramps (−100 mV to +50 mV over 500 ms) followed by 200 ms at +50 mV and repeated every 2 s. To quantify current size and time course of current amplitude, currents at +50 mV were averaged for each trace and normalized to the initial current I 0 before drug application. In cerebellar granule cells, the standing outward current, IK SO , was measured at +50 mV after 2.5 s of depolarization to minimize currents through voltage-dependent K + channels by inactivation. TIRF microscopy TIRF imaging was performed as previously described [55] . In brief, we used a BX51WI upright microscope equipped with a TIRF-condenser (Olympus, Hamburg, Germany), directing a 488-nm laser to obtain total reflection. Fluorescence images were acquired every 4 s with a 530-nm-long-pass emission filter and a CCD camera controlled by TillvisION software (TILL Photonics GmbH, Gräfelfing, Germany). Mean fluorescence intensity F of a single region of interest chosen to cover the majority of the cell’s footprint was background subtracted and normalized to the averaged intensity F 0 at the beginning of the experiment or immediately before application of the receptor agonist. FRET microscopy Fluorescence resonance energy transfer between Gα q -CFP and YFP-PLCβ3 was measured essentially as described [53] . In brief, CHO cells were transiently transfected with Gα q -CFP, YFP-PLCβ3, M1R, as well as Gβ 1 and Gγ 2 , to maintain stoichiometry of heterotrimeric G-proteins [53] . Single whole-cell patch-clamped cells were imaged on a Nikon Eclipse TE2000-U inverted microscope equipped with a Nikon Plan Apo VC 60x/1.40 Oil ∞/0.17 DIC N2 WD 0.13 oil-immersion objective (Nikon GmbH, Düsseldorf, Germany). To avoid fluorophore (YFP) quenching, intracellular chloride was reduced to 60 mM in these experiments with KCl replaced by equimolar K-Aspartate. The fluorophores were excited using an Oligochrome (Till Photonics, Gräfelfing, Germany), and fluorescence intensities were acquired with fluorescence detection unit (FDU) photodiodes and Oligochrome Imagining Control Unit (ICU FDU-2) (TILL Photonics). CFP was excited through a 430/24 ET bandpass filter. Fluorescence emission intensities were collected using a beam splitter with a 480/40m ET bandpass for CFP (F 480 ) and a 535/30m ET bandpass filter for YFP (F 535 ) (all filters from AHF Analysetechnik AG, Tübingen, Germany). FRET ratio was calculated as F 535 /F 480 from background-corrected traces and given as FRET/FRET baseline (relative FRET ratio). Oligochrome control and fluorescence intensity acquisition was performed simultaneous to voltage clamp recordings using an EPC-10 USB patch clamp amplifier in combination with PatchMaster software (HEKA Electronics, Lambrecht, Germany). Data analysis Analysis and statistical testing of electrophysiological and imaging data were performed with IGOR Pro (WaveMetrics, Lake Oswego, OR, USA). Data are shown as mean±s.e.m. with numbers in the summary graphs indicating the number of experiments (individual cells or patches). Unless indicated otherwise, the two-tailed Dunnett’s test was used for statistical testing. Asterisks denote the significance level, where *** indicates P <0.001, ** indicates P <0.01, and * indicates P <0.05. How to cite this article: Wilke, B. U. et al. Diacylglycerol mediates regulation of TASK potassium channels by Gq-coupled receptors. Nat. Commun. 5:5540 doi: 10.1038/ncomms6540 (2014).